Tumour-initiating stem-like cells in human prostate cancer exhibit increased NF-κB signalling Androgen depletion is a key strategy for treating human prostate cancer, but the presence of hormone-independent cells escaping treatment remains a major therapeutic challenge. Here, we identify a minor subset of stem-like human prostate tumour-initiating cells (TICs) that do not express prostate cancer markers, such as androgen receptor or prostate specific antigen. These TICs possess stem cell characteristics and multipotency as demonstrated by in vitro sphere-formation and in vivo tumour-initiation, respectively. The cells represent an undifferentiated subtype of basal cells and can be purified from prostate tumours based on coexpression of the human pluripotent stem cell marker TRA-1-60 with CD151 and CD166. Such triple-marker-positive TICs recapitulate the original parent tumour heterogeneity in serial xeno-transplantations indicating a tumour cell hierarchy in human prostate cancer development. These TICs exhibit increased nuclear factor-κB activity. These findings are important in understanding the molecular basis of human prostate cancer. Prostate cancer is a pressing public concern, as it has become the most common form of cancer in men in the Western world. Although androgen deprivation is a key therapeutic strategy in human prostate cancer, a small number of prostate cancer cells can thrive after anti-androgen treatment and become lethal even with castrate levels of testosterone [1] , [2] . This highlights the presence of androgen independent cells with tumour-regenerating capacity and the need for targeting them. It is well known that the normal prostate can undergo repeated cycles of castration-dependent regression and hormone-induced regrowth when supported by populations of putative prostate stem cells [3] , [4] . In normal development of the prostate gland, a subset of androgen-independent basal and/or intermediary cells can function as multipotent progenitors that give rise to androgen-dependent differentiated luminal cells [5] , [6] . Human prostate cancers may also contain rare and distinct stem-like cells responsible for tumour formation similar to those found in other cancers [7] , [8] , [9] , [10] , [11] . Multiple cell types in the prostate gland have also been considered to be potential cell(s) of origin for tumour development [12] , [13] , [14] , [15] . For example, a subset of castration-resistant postmitotic luminal cells was demonstrated to acquire proliferative capacity causing an expansion of luminal cells associated with mouse prostate tumours in a pten tumour suppressor deleted background [14] . These results were in agreement with a previously suggested dedifferentiation model of cancer cell origin [16] . However, in other studies basal epithelial stem-like cells were also shown to be efficient targets for tumour-initiation in murine prostate cancer [13] . Although these data suggest that murine prostate cancer can arise from multiple tumour cell types, the identification of specific markers for prospective isolation of precisely tumour-initiating cells (TICs) has remained an important aim in the field of human prostate cancer research. Normal and cancer stem cells were believed to express a shared set of markers [17] . However, because of their heterogeneous expression within normal and tumour tissues, many putative stem cell markers, such as CD44, CD133 and their isoforms, identify multiple cell types including sub-populations of stromal cells and interstitial cells such as immuno-stimulatory cells [2] , [16] , [18] , [19] . Moreover, in vitro cell culture conditions, in vivo tissue differentiation or exposure to cytokines affect expression of these markers and also result in considerable overlap of signalling pathways between cells that are positive and negative for these markers [20] , [21] , [22] , [23] , [24] . Therefore, identification of unique markers and signalling pathways in TICs has become an important goal for understanding the molecular basis of human prostate cancer and for developing precise therapeutic strategies in patients. In this study, we isolated TICs with stem cell-like properties from human prostate tumours. These cells are androgen receptor (AR)-negative, express TRA-1-60 and exhibit active nuclear factor κB (NF-κB) signalling. Our findings suggest that the functional NF-κB pathway may be important in maintaining the conventional therapy resistant stem-like TICs in human prostate cancer. Stem cell-like cells in human prostate tumours We investigated the human prostate TICs using the CWR22 orthotopic (OT, injection into prostate) tumour xenograft system that offers a reproducible in vivo source for providing sufficient amounts of human prostate tumour cells from a native microenvironment over successive transplantations [25] . We reasoned here that a sub-population of self-renewing stem-like prostate cancer cells is responsible for sustaining tumour growth through sequential transplantations in a manner comparable to that observed in many other human cancers [18] . We first investigated sphere-formation ability of the tumour cells as a surrogate in vitro assay for their self-renewal ability and for the retrospective identification of stem-like tumour cells [26] . We observed that dissociated tumour cells formed spheres, which we henceforth will refer to as 'primary spheres'. However, the sphere formation efficiency was very low (1–2 spheres/2,500–5,000 total tumour cells) as determined by limiting dilution assays ( Fig. 1a ). A minor subset of human patient primary prostate tumour cells also had sphere-forming ability albeit with even lower efficiency (about tenfold less). We observed a gradual increase in the total number of primary spheres formed over time for a given number of total tumour cells ( Fig. 1b ), sphere growth as determined by the increase in number of cells per sphere ( Fig. 1c ) and sphere-forming ability of serially passaged sphere cells (about 5- and 25-fold higher in secondary and tertiary sphere formation assays, respectively; Fig. 1d ). These data demonstrate differential sphere-forming abilities among various cell types in the tumour and rule out simple cell aggregation as a primary mechanism of sphere formation. Quantitative analysis of tumour-initiation efficiency through limiting dilution experiments revealed that tumour-initiation with primary sphere-cells was at least 100-times more efficient than with the total tumour cells ( Fig. 1e ). Moreover, tumour initiation at OT versus sub-cutaneous (SC)-sites was about ten-times more efficient. Unless otherwise stated, we used OT-tumour-initiation assays in all further experiments. 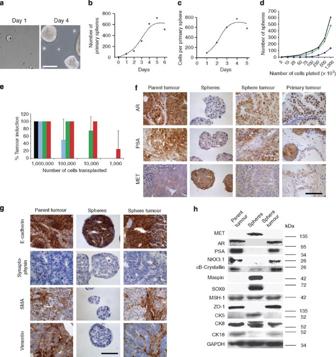Figure 1: A subset of human prostate TICs exhibits sphere-forming potential and multipotency. Unless stated otherwise, human prostate CWR22 OT-tumours were used. (a) Phase contrast images of primary sphere formation by the total tumour cells. Scale bar, 100 μm. (b) Time course of primary sphere formation (sphere number per 8×105total tumour cells plated,n=4). (c) Time course of primary sphere growth (average number of cells per primary sphere,n=4). (d) Efficiency of sequential derivation of primary (blue circle), secondary (green square) and tertiary spheres (black triangle) determined as a function of equal numbers of starting cells from total tumour, primary spheres and secondary spheres, respectively;n=4. (e) Limiting dilution experiments determining tumour-initiation efficiency (% tumour induction) at the orthotopic (blue, tumour cells; red, primary sphere cells) and subcutaneous (black, tumour cells; green, primary sphere cells) sites. Data represents the 4-week end-point results following transplantation. Mean±s.d. (n=4). (f,g) CWR22 OT-tumour (parent tumour), the tumour cell-derived primary spheres (spheres), the sphere-derived OT-tumour (sphere tumour) and human patient primary prostate tumour (primary tumour) were used for comparative immunohistochemistry (IHC). Scale bar, 50 μm. (f) Comparative IHC for expression of differentiated prostate cell markers (AR, PSA and MET) in primary spheres versus tumours. (g) Comparative IHC for expression of markers for epithelial cells (E-cadherin) versus differentiated cells in the tumour, namely neuroendocrine cells (synaptophysin), myoepithelial cells (smooth muscle actin, SMA), and mesenchymal cells (vimentin). (h) Western blots of whole cell extracts of the parent tumour, primary spheres and sphere tumour analyzing the expression of markers for prostate basal cell (CK5), luminal cell (AR, PSA, NKX3.1, CK8 and CK18), primary prostate cancer cell (MET, αB-crystallin and maspin), putative stem cell (Musashi-1, MSH-1), basal epithelial stem cell (SOX9), cell polarity/differentiation (ZO-1) and loading control (glyceraldehyde 3-phosphate dehydrogenase, GAPDH). Figure 1: A subset of human prostate TICs exhibits sphere-forming potential and multipotency. Unless stated otherwise, human prostate CWR22 OT-tumours were used. ( a ) Phase contrast images of primary sphere formation by the total tumour cells. Scale bar, 100 μm. ( b ) Time course of primary sphere formation (sphere number per 8×10 5 total tumour cells plated, n =4). ( c ) Time course of primary sphere growth (average number of cells per primary sphere, n =4). ( d ) Efficiency of sequential derivation of primary (blue circle), secondary (green square) and tertiary spheres (black triangle) determined as a function of equal numbers of starting cells from total tumour, primary spheres and secondary spheres, respectively; n =4. ( e ) Limiting dilution experiments determining tumour-initiation efficiency (% tumour induction) at the orthotopic (blue, tumour cells; red, primary sphere cells) and subcutaneous (black, tumour cells; green, primary sphere cells) sites. Data represents the 4-week end-point results following transplantation. Mean±s.d. ( n =4). ( f , g ) CWR22 OT-tumour (parent tumour), the tumour cell-derived primary spheres (spheres), the sphere-derived OT-tumour (sphere tumour) and human patient primary prostate tumour (primary tumour) were used for comparative immunohistochemistry (IHC). Scale bar, 50 μm. ( f ) Comparative IHC for expression of differentiated prostate cell markers (AR, PSA and MET) in primary spheres versus tumours. ( g ) Comparative IHC for expression of markers for epithelial cells (E-cadherin) versus differentiated cells in the tumour, namely neuroendocrine cells (synaptophysin), myoepithelial cells (smooth muscle actin, SMA), and mesenchymal cells (vimentin). ( h ) Western blots of whole cell extracts of the parent tumour, primary spheres and sphere tumour analyzing the expression of markers for prostate basal cell (CK5), luminal cell (AR, PSA, NKX3.1, CK8 and CK18), primary prostate cancer cell (MET, αB-crystallin and maspin), putative stem cell (Musashi-1, MSH-1), basal epithelial stem cell (SOX9), cell polarity/differentiation (ZO-1) and loading control (glyceraldehyde 3-phosphate dehydrogenase, GAPDH). Full size image The stem-like TICs do not express androgen receptor and prostate-specific antigen The spheres express distinct characteristics and are multipotent as the sphere-cell-derived tumours (sphere tumours) reconstituted histopathological features and immunophenotypes of the original OT-human prostate CWR22 tumour (parent tumour) and closely mimicked the features of freshly obtained patient prostate tumour specimens (primary tumours; Fig. 1f–h ; Supplementary Fig. S1a–d ). Thus, these stem-like sphere cells do not express key markers of prostate cancer, including AR, prostate specific antigen (PSA), NKX3.1 (androgen/AR-regulated transcriptional coactivator) and cytokeratin-18 (CK18, differentiated luminal cell enriched marker). In contrast, cancer stem cell and cell-proliferation-associated markers MET receptor kinase, Musashi-1, inhibitor of differentiation 1, phospho-histone 3 and Ki67 are selectively enriched in these spheres relative to tumours. We also found that the AR-/PSA-negative stem-like sphere cells are of basal epithelial-like cell type based on the expression of E-cadherin, cytokeratin-5 (CK5) and SOX9 and lack of expression of markers of myoepithelial cells (smooth muscle actin), mesenchymal cells (vimentin) and neuroendocrine cells (synaptophysin). However, these sphere cells also lack detectable expression of basal cell enriched, p63 and its polarity associated, zonula occludens-1 (ZO-1). Thus, these sphere-forming TICs represent a distinct cancer stem-like cell compartment in the human prostate tumour. Human prostate TICs express novel pluripotent cell markers By fluorescence-activated cell sorting (FACS), we investigated novel cell surface marker expression that could facilitate prospective isolation of the TICs in the human prostate CWR22 OT-tumours. First, we confirmed the expression of a set of markers known to associate with stem-like tumour cells in other epithelial cancers, including human prostate tumours [17] , [27] . They included epithelial cellular adhesion molecule (EpCAM), hyaluronic acid receptor (CD44) and integrins (α2-integrin, α6-integrin and β4-integrin; Fig. 2a ). Prostate tumour cells expressing these markers displayed increased sphere-formation capacity as compared with unsorted total tumour cells or cells expressing β4-integrin ( Fig. 2b ). Except for CD44, the percentage of cells expressing these markers (EpCAM, α2-integrin for example) was consistently enriched over sequential passages of sphere cells. The above markers are associated with many different cell types including stromal and/or interstitial cells in the prostate and in other organs. Therefore, to facilitate precise identification of stem-like TICs, we investigated novel markers such as the tumour rejection antigen, TRA-1-60, a cell surface epitope of human embryonic, embryonal germline and teratocarcinoma stem cells [28] . Sphere-forming cells and a subset of tumour cells express TRA-1-60, related pluripotent stem cell markers such as TRA-1-81 and stage-specific embryonic antigens such as SSEA1, SSEA4 for example ( Fig. 2a, c–f ; Supplementary Fig. S2 ). TRA-1-60 or TRA-1-81-positive tumour cells formed spheres more efficiently than cells positive for other known markers ( Fig. 2b,g ), and the TRA-1-60-positive tumour cells were moderately more efficient in tumour induction than the primary sphere cells ( Fig. 3a ). 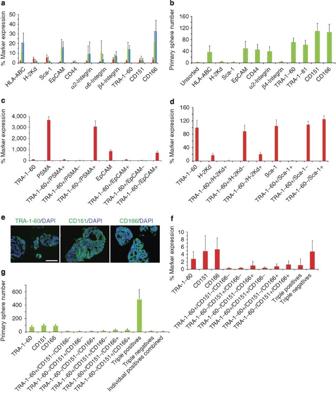Figure 2: Prospective isolation and characterization of human prostate TICs. (a) Percent marker expression in parent tumours (red) or the sequentially derived primary (green) and secondary (blue) spheres. Mean±s.d. (n=10). (b) Primary sphere formation is affected by the markers expressed in tumour cells (primary spheres/5,000 tumour cells). Mean±s.d. (n=10). (c,d) Percent coexpression of TRA-1-60 and (c) human-specific-PSMA or -EpCAM or (d) mouse-specific MHC Class I H-2KD or -Sca-1 in tumour cells. Mean±s.d. (n=4). (e) Immunofluorescence labelling of TRA-1-60, CD151 and CD166 in primary spheres and 4′-6-diamidino-2-phenylindole (DAPI) represents counterstain. Scale bar, 50 μm. (f) Percent combinatorial expression of the triple-markers in tumour cells. Mean±s.d. (n=8). (g) Marker-specific primary sphere-formation efficiency (determined as above inb). Mean±s.d. (n=5). Figure 2: Prospective isolation and characterization of human prostate TICs. ( a ) Percent marker expression in parent tumours (red) or the sequentially derived primary (green) and secondary (blue) spheres. Mean±s.d. ( n =10). ( b ) Primary sphere formation is affected by the markers expressed in tumour cells (primary spheres/5,000 tumour cells). Mean±s.d. ( n =10). ( c , d ) Percent coexpression of TRA-1-60 and ( c ) human-specific-PSMA or -EpCAM or ( d ) mouse-specific MHC Class I H-2KD or -Sca-1 in tumour cells. Mean±s.d. ( n =4). ( e ) Immunofluorescence labelling of TRA-1-60, CD151 and CD166 in primary spheres and 4′-6-diamidino-2-phenylindole (DAPI) represents counterstain. Scale bar, 50 μm. ( f ) Percent combinatorial expression of the triple-markers in tumour cells. Mean±s.d. ( n =8). ( g ) Marker-specific primary sphere-formation efficiency (determined as above in b ). Mean±s.d. ( n =5). 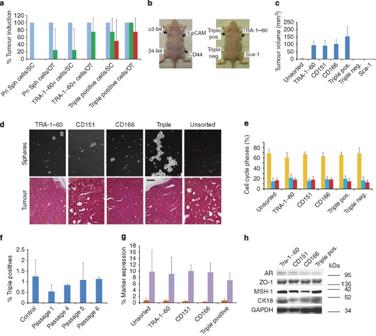Figure 3:In vivotumour-initiation by purified human prostate TICs. (a) Limiting dilution experiments for determining percent tumour-initiation by equal numbers of sphere cells, TRA-1-60-positive cells or triple positives transplanted at OT or SC sites. Blue, 10,000 cells; green, 1,000 cells and red, 200 cells. Data represents the 4-week end-point results following transplantation. (b–h) Unless otherwise stated, 5,000 marker-positive or total tumour (unsorted control) cells were used per transplantation. (b) Representative SC tumour growth at 5 weeks following transplantation. Unsorted represents a control tumour-derived from transplantation of 2×106total tumour cells. (c) Tumour-initiation efficiency (represented as tumour volume) of the marker-positive cells at 5 weeks following transplantation. (d) Upper panel: Dark field images of primary spheres formed by marker-positive cells. Lower panel: hematoxylin and eosin staining of tumours derived from different marker-positive tumour cells. Scale bar, 100 μm. (e) Relative levels of G1 (yellow), G2 (blue) and S (red) phases of cell cycle in the different marker-positive tumour cells. Unsorted represents total tumour cells. (f) Percent triple-marker expression in sequentially passaged OT-tumours that were initially derived from the triple-marker-positive tumour cells. Percentage triple-marker-positive cells in the parent tumour form the control. (g) Maintenance of triple-marker-positive cells in the secondary passaged tumours derived from indicated marker-specific primary tumour cells. Unsorted is as described in (b). Orange-triple-marker-positive cells and purple-triple-marker-negative cells. (h) Immunoblot analysis of whole cell extracts of the tumours derived from marker-positive tumour cells. Glyceraldehyde 3-phosphate dehydrogenase (GAPDH) represents the loading control. Mean±s.d.,n≥3. Full size image Figure 3: In vivo tumour-initiation by purified human prostate TICs. ( a ) Limiting dilution experiments for determining percent tumour-initiation by equal numbers of sphere cells, TRA-1-60-positive cells or triple positives transplanted at OT or SC sites. Blue, 10,000 cells; green, 1,000 cells and red, 200 cells. Data represents the 4-week end-point results following transplantation. ( b – h ) Unless otherwise stated, 5,000 marker-positive or total tumour (unsorted control) cells were used per transplantation. ( b ) Representative SC tumour growth at 5 weeks following transplantation. Unsorted represents a control tumour-derived from transplantation of 2×10 6 total tumour cells. ( c ) Tumour-initiation efficiency (represented as tumour volume) of the marker-positive cells at 5 weeks following transplantation. ( d ) Upper panel: Dark field images of primary spheres formed by marker-positive cells. Lower panel: hematoxylin and eosin staining of tumours derived from different marker-positive tumour cells. Scale bar, 100 μm. ( e ) Relative levels of G1 (yellow), G2 (blue) and S (red) phases of cell cycle in the different marker-positive tumour cells. Unsorted represents total tumour cells. ( f ) Percent triple-marker expression in sequentially passaged OT-tumours that were initially derived from the triple-marker-positive tumour cells. Percentage triple-marker-positive cells in the parent tumour form the control. ( g ) Maintenance of triple-marker-positive cells in the secondary passaged tumours derived from indicated marker-specific primary tumour cells. Unsorted is as described in ( b ). Orange-triple-marker-positive cells and purple-triple-marker-negative cells. ( h ) Immunoblot analysis of whole cell extracts of the tumours derived from marker-positive tumour cells. Glyceraldehyde 3-phosphate dehydrogenase (GAPDH) represents the loading control. Mean±s.d., n ≥3. Full size image Mouse OT xenografts of human prostate tumour tissue contain a mixed population of cells expressing both human and mouse antigens. Therefore, we verified that expression of human-specific epitopes, such as major histocompatibility complex (MHC) HLA-Class I ABC, but not mouse-specific antigen MHC Class I H-2K d and stem cell antigen-1 (Sca-1), in the tumour cells was correlated with their sphere-formation ( Fig. 2a,b ) and tumour initiation ( Table 1 ) abilities. Moreover, the TRA-1-60-positive cells also express the human-specific-EpCAM, as well as -PSMA epitopes ( Fig. 2c ), whereas the tumour cells double positive for expression of TRA-1-60 and mouse specific Sca-1 or H-2K d were not found ( Fig. 2d ). This indicates that the sphere-forming and tumour-initiating TRA-1-60-positive cells represent epithelial cells of human prostate cell origin. Table 1 Tumour initiation by sphere cells and purified tumour cells. Full size table Next, we investigated the expression of additional markers such as CD166 and CD151, which are known to associate with colon epithelial cancer stem cells [29] and other stem-like cells in tumour stroma, respectively, and during prostate cancer progression [30] ( Supplementary Fig. S2 ). Tumour cells expressing CD151 or CD166 exhibited greater efficiency in sphere formation than any of the above tested markers ( Fig. 2a,b ) and immunofluorescence verified their expression in spheres, akin to that of TRA-1-60 ( Fig. 2e ). Sphere-forming and tumour-initiation abilities were significantly diminished in cells sorting negative for expression of TRA-1-60, CD151 or CD166 ( Figs 2g , 3b,c ; Table 1 ). We also tested for combinatorial expression of the above three markers ( Supplementary Figs S3 and S4 ), and identified a minor triple-marker-positive subset (TRA-1-60+CD151+CD166+ cells) among various sub-populations of cells expressing other possible marker combinations ( Fig. 2f ). The triple-marker-positive cells had considerably higher sphere-forming ability than the single or double positives and triple negatives ( Fig. 2g ). The sphere-forming ability could not be enhanced even after combining all three individual subsets of cells exclusively expressing one of the above three markers suggesting that coexpression of the three markers reflects a hierarchical organization of sphere formation propensity in the prostate tumour cells. Limiting dilution studies revealed that prospectively purified triple-marker-positive cells reproducibly formed tumours at OT and SC locations with at least fivefold more efficiency than those formed with the TRA-1-60-positive cells ( Fig. 3a ). When compared with an equal number of cells-positive for gross expression of any of the above markers, the triple-marker-positive cells induced increased tumour growth ( Fig. 3b,c ) and enhanced onset of tumour-initiation ( Table 1 ). Similar to the data on sphere formation, cells exclusively positive for any one or two of the three markers (but negative for the remaining marker(s)), unsorted single cells derived from tumour, human β4-integrin-positive cells or mouse-specific MHC Class I H-2Kd- and Sca-1-positive cells served as negative controls in the tumour-initiation experiments. Human prostate non-tumourigenic epithelial cells obtained from two independent sources (PrEC from Lonza and RWPE1 from American Type Culture Collection) also did not initiate tumour formation under these conditions ( Table 1 ). Interestingly, tumours derived from various marker-positive tumour cells with different sphere-forming efficiencies or unfractionated total tumour cells ( Fig. 3d ) displayed comparable histopathological features ( Fig. 3d ) with comparable levels of cell cycle phases ( Fig. 3e ). Tumour derived from triple-marker-positive cells could be serially passaged in vivo (at least six passages) without obvious changes in percentage of marker-positive cells ( Fig. 3f ). Tumours induced from single marker-positive cells gave rise to both marker-positive and -negative cells ( Fig. 3g ) and showed biochemical marker expression profiles ( Fig. 3h ) similar to those observed in parent tumours ( Fig. 1h ). These results also suggest that the triple-marker-positive cells both self-renew and differentiate by recapitulating a cellular hierarchy of the original parent tumour. The triple-marker expression and the association with tumour-initiation were consistent in additional human prostate cancer cell line-derived xenograft tumour models, namely, androgen-independent metastatic prostate cancer cell line-derived DU-145 (brain metastasis), PC3 (bone metastasis) and VCaP (vertebral metastasis) xenograft tumours, and also in another androgen-dependent and human patient-derived primary OT-xenograft tumour (PC-82; Table 2 ; Supplementary Fig. S5 ). All the resulting tumours exhibited their expected immunohistochemical characteristics ( Fig. 4a ) such as cytosolic localization of AR in androgen-insensitive DU-145 and PC3 tumours, or nuclear localization in androgen-sensitive VCaP and PC-82 tumours. All these tumours contained a set of triple-marker-positive cells ( Table 2 ). Tumours derived from triple-marker-positive DU-145 tumour cells were sequentially passaged in vivo over multiple transplantation cycles ( Fig. 4b ). The marker-positive cells from the DU-145 tumour recapitulated the original parent tumour heterogeneity by hierarchically differeniating in vivo into both marker-positive and -negative tumour cells. Marker expression and sphere-forming/tumour-initiating abilities were also correlated in the DU-145 tumour cells, although the marker negative cells have considerably diminished sphere-forming and tumour-initiating abilities ( Fig. 4c,d ). We next verified the expression of each of these triple-markers in freshly resected human patient specimens from prostate tumour by immunofluorescence ( Fig. 4e ) and FACS ( Fig. 4f ) or from other epithelial tumours of breast, colon and ovary by FACS ( Fig. 4g ). Cells positive for expression of the TRA-1-60 and triple-marker-positive cells were enriched in other epithelial tumour specimens when compared with the respective patient-matched normal tissues. Table 2 Percent marker-positive cells in various human prostate tumours. 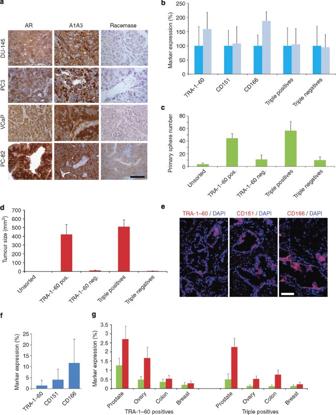Figure 4: Triple-marker expression in other prostate tumours and patient specimens. (a) Comparative immunohistochemical characterization of DU-145, PC3, VCaP and PC-82 tumours. Scale bar, 50 μm. (b) Percent marker-positive cells maintained after sequentialin vivopassages of DU-145 tumours that were initially derived from the triple-marker-positive cells. Blue, passage1 and light blue, passage2. Mean±s.d. (n=4). (c)In vitroprimary sphere-formation and (d)In vivotumour initiation. Prospectively isolated 2,500 marker-positive DU-145 tumour cells were used. Tumour size was determined as tumour volume. Mean±s.d. (n=4). Unsorted control represents single cells of tumour. (e) Immunofluorescence labelling of markers in fresh frozen human patient primary prostate tumour specimens, with 4′-6-diamidino-2-phenylindole (DAPI) counterstain. Scale bar, 100 μm. (f) Percent marker-positive cells in human patients' prostate tumour specimens. Mean±s.d. (n=6). (g) Percent marker-positive cells in a variety of epithelial tumour specimens from clinical patients. Red, tumour cells and green, patient-matched normal tissue cells. Mean±s.d. (n=3). Full size table Figure 4: Triple-marker expression in other prostate tumours and patient specimens. ( a ) Comparative immunohistochemical characterization of DU-145, PC3, VCaP and PC-82 tumours. Scale bar, 50 μm. ( b ) Percent marker-positive cells maintained after sequential in vivo passages of DU-145 tumours that were initially derived from the triple-marker-positive cells. Blue, passage1 and light blue, passage2. Mean±s.d. ( n =4). ( c ) In vitro primary sphere-formation and ( d ) In vivo tumour initiation. Prospectively isolated 2,500 marker-positive DU-145 tumour cells were used. Tumour size was determined as tumour volume. Mean±s.d. ( n =4). Unsorted control represents single cells of tumour. ( e ) Immunofluorescence labelling of markers in fresh frozen human patient primary prostate tumour specimens, with 4′-6-diamidino-2-phenylindole (DAPI) counterstain. Scale bar, 100 μm. ( f ) Percent marker-positive cells in human patients' prostate tumour specimens. Mean±s.d. ( n =6). ( g ) Percent marker-positive cells in a variety of epithelial tumour specimens from clinical patients. Red, tumour cells and green, patient-matched normal tissue cells. Mean±s.d. ( n =3). Full size image Global gene expression in stem-like human prostate TICs To gain molecular insights into the potential mechanism(s) behind the functional correlation between cell surface markers expression and their sphere-/tumour-forming efficiency (S/TFE), we determined global expression patterns of both mRNAs and microRNAs (miRNAs) from the same marker-positive cells. We classified the resulting data into three sets based on their marker-specific functional S/TFEs: (a) high S/TFE set (representing the triple-marker-positive tumour cells that coexpress TRA-1-60, CD151 and CD166; n =3), (b) moderate S/TFE set (representing tumour cells positive for gross expression of TRA-1-60, CD151 or CD166; n =7) and (c) low S/TFE set (representing tumour cells positive for gross expression of α2-integrin, EpCAM or CD44; n =3). The above data sets were paired against the controls derived from unsorted matched tumour cells ( n =6) or cells positive for expression of β4-integrins. Expression of a set of mRNAs was shared in all the S/TFE data sets ( Fig. 5a ). In contrast, only a few shared miRNAs were observed among all three S/TFE data sets ( Supplementary Fig. S6a ). But a relatively large list of miRNAs was common between moderate and high S/TFE data sets. Gene expression data analysis using DAVID [31] ( http://david.abcc.ncifcrf.gov ) and gene ontology revealed a striking enrichment in gene expression related to cell development, differentiation and cell death ( Fig. 5b ). Importantly, an involvement of protein kinase C (PKC)/NF-κB signalling axis was evident in all the mRNA data sets (as exemplified by NFKBIA, LGALS1, CRYAB (αB-crystallin), IFIH1, CGB5, CGB8, XM_938419, NRAP, PTPLAD2, TSHZ1; Fig. 5c–f ) and the miRNA data sets ( Supplementary Fig. S6b–e ) in addition to those related to stem cell biology, embryonic development and oncogenesis. 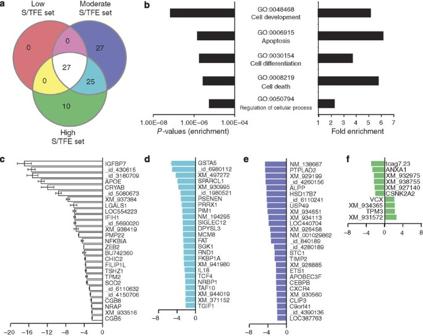Figure 5: Global mRNA expression in marker-positive human prostate tumour cells. (a) Venn-diagram of genes differentially expressed in prospectively isolated CWR22 OT-tumour cells with low (expressing EpCAM, CD44 or α2-integrin), moderate (expressing TRA-1-60, CD151 or CD166) and high (triple-marker-positives) sphere/tumour-forming efficiencies (S/TFE). Gene expression data in β4-integrin-positive (no sphere-forming) cells and the total tumour cells were used as baseline expression control. (b) Fold enrichment of gene ontology based functional categories in all the S/TFE data sets. (c–f) Catalogue of top differentially expressed genes: (c) shared among all the above three data sets, (d) shared between moderate and high S/TFE data sets, (e) expressed specifically in moderate S/TFE data set and (f) expressed specifically in high S/TFE data set. Figure 5: Global mRNA expression in marker-positive human prostate tumour cells. ( a ) Venn-diagram of genes differentially expressed in prospectively isolated CWR22 OT-tumour cells with low (expressing EpCAM, CD44 or α2-integrin), moderate (expressing TRA-1-60, CD151 or CD166) and high (triple-marker-positives) sphere/tumour-forming efficiencies (S/TFE). Gene expression data in β4-integrin-positive (no sphere-forming) cells and the total tumour cells were used as baseline expression control. ( b ) Fold enrichment of gene ontology based functional categories in all the S/TFE data sets. ( c – f ) Catalogue of top differentially expressed genes: ( c ) shared among all the above three data sets, ( d ) shared between moderate and high S/TFE data sets, ( e ) expressed specifically in moderate S/TFE data set and ( f ) expressed specifically in high S/TFE data set. Full size image Constitutive NF-κB signalling and function in the stem-like TICs We investigated the differences between the TRA-1-60-positive spheres with tumour-initiating potential and tumours with regards to various signalling pathways mediated by canonical receptor tyrosine kinase, insulin, AKT, ERK and Wnt (for example, β-catenin expression). Except for a diminished level of insulin growth factor receptor 1β phosphorylation in the spheres ( Fig. 6a ; Supplementary Fig. S1a,b,d ), there were no considerable differences in the activation of conventionally studied signalling pathway components. Therefore, we reasoned from genome-wide expression data that constitutively active PKC/NF-κB pathway may be functionally associated with the stem-like human prostate TICs. We verified that a classical PKC (PKC α) was specifically activated in the stem-like TICs by immunoblotting for PKC α protein phosphorylation ( Fig. 6a ). However, levels of other PKCs (pan-phosphorylated PKCβII and atypical PKCs, PKC ζ/λ) remained unaffected, whereas the PKD or PKCμ remained moderately lower in the sphere cells as compared with the tumour cells. Next, we confirmed the microarray data on downregulation of transcription of NFKBIA ( Fig. 5c ) with a specific decrease in its protein level, by including the other positive controls such as IGFBP7 and αB-crystallin ( Figs 1h and 6a ). There was also an increased accumulation of NF-κB p65 and its K310 acetylated form specifically nuclear localized in the spheres ( Fig. 6b ), implying a potential functional importance of sustained NF-κB signalling, as deacetylation of NF-κB p65 was previously shown to inhibit its transcriptional activity and induce cellular apoptosis [32] . Furthermore, the sphere cells showed increased levels of a proinflammatory cytokine interleukin 6 (IL-6), the anti-apoptotic Bcl-2 family member human myeloid cell leukemia-1 (MCL-1) and additional regulators of epithelial cell proliferation and apoptosis, such as 14-3-3σ ( Fig. 6a,c ). 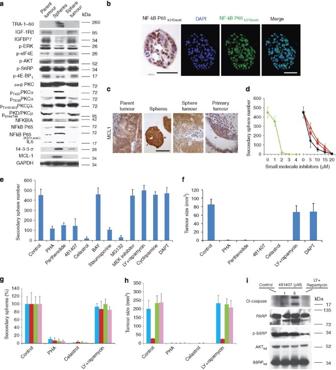Figure 6: NF-κB-signalling in stem-like human prostate TICs. Western blots of whole cell extracts of the parent tumour, spheres and the sphere tumour analyzing (a) various signalling pathway components, with glyceraldehyde 3-phosphate dehydrogenase (GAPDH) representing loading control. (b) Nuclear localization of NF-κB in stem-like sphere-forming cells. Immunofluorescence (scale bar, 100 μm) or immunohistochemistry (scale bar, 50 μm) of acetylated (K310) NF-κB visualized in the nucleus and counterstained by DAPI (IF) or hematoxylin (IHC). (c) Comparative immuno-histochemical analysis of MCL-1 expression in primary spheres versus the parent tumour, sphere tumour and human patient primary tumour. Scale bar, 100 μm. (d) Dose-dependent effects of small molecule inhibitors on secondary sphere formation. Inhibitors were administered to primary sphere-forming total tumour cells. Red, PHA (PHA 665752); brown, parthenolide; black, 481407; green, celastrol. (e) Preliminary screening to test effect of inhibitors of different signalling pathways on secondary sphere-formationin vitro. PHA (10ìμM), parthenolide (10ìM), 481407(5ìM), celastrol (2ìM), BAY (BAY11-7082, 10ìM), staurosporine (0.05ìM), MG132 (0.5ìM), LY (LY294002, 10ìM) + rapamycin (20nM), cyclopamine (2ìM) or DAPT (10ìM) were administered, wherein the control represents dimethylsulphoxide (DMSO)-treated set. (f) Primary sphere-forming tumour cells were treated with the inhibitors of MET (PHA: 20 μM), activated NF-κB signalling, (parthenolide: 20 μM; 481407: 20 μM; celastrol: 3 μM), PI3 kinase signalling (LY 294002: 15 μM)+mTOR signalling (rapamycin: 40nM) or Notch signalling (DAPT: 20 μM) were xeno-transplanted subcutaneously. Tumour size was determined by tumour volume at the 5-week end point. (g,h) Effects of these signalling inhibitors on secondary sphere formation (g) and tumour-initiation (h) across multiple human prostate tumour xenograft models. Same number of total tumour cells from human prostate DU-145 SC-(blue)/ PC-82 OT-(red) tumours or prospectively purified TRA-1-60-positive cells from the CWR22 OT-(green)/DU-145 SC-(pink) tumours were used. Tumour size was determined as above. (i) Immunoblot analyses of cleared caspase (Cl-caspase) and PARP cleavage in the primary spheres following administration of NF-κB and AKT/mTOR signalling inhibitors. Whole cell extracts prepared 6 h-post drug administration were analysed by western blotting. Control represents DMSO-treated set, whereas the total AKT and total S6RP levels served as loading controls. Mean±s.d.,n≥4. Figure 6: NF-κB-signalling in stem-like human prostate TICs. Western blots of whole cell extracts of the parent tumour, spheres and the sphere tumour analyzing ( a ) various signalling pathway components, with glyceraldehyde 3-phosphate dehydrogenase (GAPDH) representing loading control. ( b ) Nuclear localization of NF-κB in stem-like sphere-forming cells. Immunofluorescence (scale bar, 100 μm) or immunohistochemistry (scale bar, 50 μm) of acetylated (K310) NF-κB visualized in the nucleus and counterstained by DAPI (IF) or hematoxylin (IHC). ( c ) Comparative immuno-histochemical analysis of MCL-1 expression in primary spheres versus the parent tumour, sphere tumour and human patient primary tumour. Scale bar, 100 μm. ( d ) Dose-dependent effects of small molecule inhibitors on secondary sphere formation. Inhibitors were administered to primary sphere-forming total tumour cells. Red, PHA (PHA 665752); brown, parthenolide; black, 481407; green, celastrol. ( e ) Preliminary screening to test effect of inhibitors of different signalling pathways on secondary sphere-formation in vitro . PHA (10ìμM), parthenolide (10ìM), 481407(5ìM), celastrol (2ìM), BAY (BAY11-7082, 10ìM), staurosporine (0.05ìM), MG132 (0.5ìM), LY (LY294002, 10ìM) + rapamycin (20nM), cyclopamine (2ìM) or DAPT (10ìM) were administered, wherein the control represents dimethylsulphoxide (DMSO)-treated set. ( f ) Primary sphere-forming tumour cells were treated with the inhibitors of MET (PHA: 20 μM), activated NF-κB signalling, (parthenolide: 20 μM; 481407: 20 μM; celastrol: 3 μM), PI3 kinase signalling (LY 294002: 15 μM)+mTOR signalling (rapamycin: 40nM) or Notch signalling (DAPT: 20 μM) were xeno-transplanted subcutaneously. Tumour size was determined by tumour volume at the 5-week end point. ( g , h ) Effects of these signalling inhibitors on secondary sphere formation ( g ) and tumour-initiation ( h ) across multiple human prostate tumour xenograft models. Same number of total tumour cells from human prostate DU-145 SC-(blue)/ PC-82 OT-(red) tumours or prospectively purified TRA-1-60-positive cells from the CWR22 OT-(green)/DU-145 SC-(pink) tumours were used. Tumour size was determined as above. ( i ) Immunoblot analyses of cleared caspase (Cl-caspase) and PARP cleavage in the primary spheres following administration of NF-κB and AKT/mTOR signalling inhibitors. Whole cell extracts prepared 6 h-post drug administration were analysed by western blotting. Control represents DMSO-treated set, whereas the total AKT and total S6RP levels served as loading controls. Mean±s.d., n ≥4. Full size image We additionally exploited the in vitro secondary sphere-formation assay to investigate the functional effects of various signalling pathway inhibitors on the primary sphere-forming TICs. Administration of MET inhibitor (PHA: PHA 665752) and NF-κB activation inhibitors (481407 compound, parthenolide and celastrol) inhibited secondary sphere formation in a dose-dependent manner ( Fig. 6d ). Similar to the activation inhibitors of NF-κB, other pharmacological inhibitors of NF-κB (MG 132, functioning at the level of proteasomes inhibition) and PKC (such as staurosporine), but not the IkBα phosphorylation inhibitor (BAY 11-7085, as expected from the lack of NFKBIA in the spheres) abrogated the secondary sphere-formation ability ( Fig. 6e ). Inhibitors of phosphoinositide-3-kinase and mTOR (LY294002 and rapamycin, respectively), hedgehog (cyclopamine), γ-secretase/Notch (DAPT) and MAP kinase kinases (MEK inhibitor: U0126) also did not affect secondary sphere formation ( Fig. 6e ). The specific inhibitory effect of NF-κB activation inhibitors on primary sphere cells' ability to form secondary spheres also correlated with a functional inhibition of tumour-initiation (measured by tumour volume; Fig. 6f ). Administration of the MET receptor inhibitor PHA and the NF-κB activation inhibitor celastrol to primary sphere-forming cells of DU-145 and PC-82 OT-tumours also inhibited their ability for in vitro secondary sphere formation ( Fig. 6g ) and in vivo tumour-initiation ( Fig. 6h ). Importantly, administration of these inhibitors to the prospectively purified primary sphere-forming TRA-1-60-positive cells of the various human prostate tumours mentioned above similarly inhibited secondary sphere-formation in cultures and tumour-initiation in animals. Finally, we confirmed that the activation inhibitor of NF-κB, 481407 induced apoptosis as determined by the accumulation of cleaved caspase and by poly ADP ribose polymerase (PARP) cleavage ( Fig. 6i ). Under these conditions, neither the activation of AKT kinase (measured as phospho-AKT levels) nor its downstream signalling (phosphorylation of S6 ribosomal protein (S6RP)), is affected, demonstrating a specificity of this drug for inducing apoptosis in NF-κB activated stem-like TICs. In contrast, LY294002 and rapamycin inhibited the phosphorylation of S6RP as expected, without inducing apoptosis as determined by the lack of accumulation of cleaved caspase and PARP cleavage products. The precise cell type(s) responsible for development of human prostate cancer and the mechanism(s) behind the resistance against traditional prostate cancer therapies in patients remain elusive. This study identifies a subset of AR-/PSA-negative human prostate tumour cells, which have stem-like cell characteristics and are efficient TICs. On the other hand, these stem-like TICs express MET, CK5 and SOX9, which characterize them as being more stem-like basal cells than differentiated luminal cells in the prostate. However, little or no expression of Nkx3.1, ZO-1, CK18 and p63 also identifies them as a largely undifferentiated and nonpolarized subset of basal cells and compares them to adult prostate stem cells localized in the basal epithelial cell compartment of the normal gland [27] , [33] . The lack of p63 expression in the basal cell-like sphere cells is also consistent with previous data on the presence of a p63-negative, stem-like subset of basal cells in the prostate gland [34] and the androgen-dependent regeneration of hormone refractory regressed p63−/− prostate [35] . A key function of basal cells with CK5+/p63– phenotype was found in prostate cancer development [5] . Enhanced expression of Ki67 (a proliferating cell marker) and weak expression of differentiated epithelial tumour cell (including prostate) marker, α-B-crystallin, in the sphere cells ( Fig. 1h ) further defines them as stem-like proliferating cancer cells. However, expression of at least one luminal cell-specific marker, cytokeratin-8 (CK8) in these stem-like TICs characterizes them as a distinct subset of basal cells with a cytokeratin expression pattern intermediate between CK5-positive basal cells and CK18-positive luminal cells. Similarly, intermediate cell types have been implicated in the growth of prostate or invasive prostate carcinoma [5] , [36] , [37] , and these cell types were also shown to express high levels of MET receptor [38] . Although MET is expressed in prostate basal epithelial cells [39] and stem cells associated with cancers [40] , overexpression of human MET was shown to have an important role in cellular transformation, and to indicate poor prognoses of a variety of epithelial cancers in patients. The inverse relationship between the expression levels of MET receptor and AR in sphere-forming TICs is consistent with previous reports on cellular transformation and androgen-independent prostate cancer growth [41] , [42] . Sox9 is known to have a role in maintaining the committed stem cell compartment by regulating AR levels and cell proliferation rates [43] . Recently, the inducible lineage-marking experiments revealed that a rare population of castration resistant Nkx3.1 positive luminal cells (although negative for expression of basal cell markers) induced prostate cancer in a mouse model of conditional Pten tumour suppressor gene deletion [14] . However, in a comparable activated AKT signalling background, prospectively isolated mouse prostate basal cells induced tumours more efficiently than their luminal cell counterparts [13] . Our data on human prostate tumours suggests that this subset of undifferentiated stem-like basal cells may represent at least one subtype of cancer stem-like cells. It is possible that there may be more than a single stem-like TIC type, and that multiple stem-like cell characteristics reflect differential activation of various oncogenic signalling pathways in the context of complex cancer cell paradigms [7] , [8] , [9] , [10] . Thus, even from the point of view of therapy development, it becomes important to precisely discriminate the cell type of origin in any given tumour. A very recent report corroborates our data, suggesting that in a transgenically manipulated oncogene-induced tumour paradigm, only basal, and not luminal, cells isolated from radical proctectomy patient specimens are capable of tumour induction on xenotransplantation [44] . Together, our data unveils a largely undifferentiated subtype of human prostate TICs with the AR−/PSA−/NKX3.1−/SOX9+/p63−/CK5+/CK8+/CK18− phenotype. Interestingly, in comparison with the total tumour cells, the TICs showed no substantial differences in expression levels of cancer-associated canonical receptor tyrosine kinases and/or their associated/downstream signalling components ( Fig. 6a ; Supplementary Fig. S1a,b,d ). The specific activation of PKCα/NF-κB signalling in stem-like human prostate TICs is consistent with the previous findings that phosphorylated forms of classical PKCs (such as PKCα) and the downstream novel PKCs mediate activation of NF-κB signalling [45] . These conditions may have affected normal NF-κB homeostasis [46] in the stem-like TICs to result in constitutive activation of NF-κB, which in turn regulates a battery of genes associated with apoptosis and tumourigenesis, as deduced from the global gene expression data. The genomic expression data as well as subsequent biochemical data-driven delineation of NF-κB signalling axis involving the IL-6/MCL-1 in the functional stem-like TICs was consistent with other relevant findings such as IL-6 (a NF-κB target) regulation of MCL-1 expression and mediation of cell survival responses by blocking apoptosis during late stage prostate carcinoma [47] , [48] , or activation of NF-κB via a positive feedback loop to maintain neoplastic transformation in a cell culture model system [49] . Moreover, involvement of NF-κB-dependent cell survival signalling was also implicated in downregulation of AR expression by the activated PKC pathways [50] and there was a mutual transcriptional interference between the expression of NF-κB p65 and AR [51] . Our results also support the contention that the activated PKCα/NF-κB pathway could have resulted in the observed lack of AR accumulation in the stem-like human prostate TICs. Although previous studies suggest a functional role of NF-κB signalling in different clonally-derived in vitro cultured tumour cells (for example, both in CD133-positive [24] and -negative [23] human prostate tumour cell cultures), epigenetically transformed cell lines [49] and in mutant-KRAS animal tumour models [52] , our data reveals for the first time a specifically increased and functional NF-κB signalling in the prospectively purified naïve stem-like human prostate TICs. A strong correlation was also found between positive NF-κB nuclear staining in patients' radical prostatectomy specimens with positive margin prostate cancer and a several-fold increase in their risk for biochemical recurrence of this disease [53] . Furthermore, our inhibitor screening data is corroborated by recent hierarchical clustering of multi-marker immunohistochemical analyses on the prognostic significance of human prostate cancer [54] , which revealed that nuclear NF-κB, but not phospho-AKT, was associated with biochemical recurrence of this disease in radical prostatectomy patients. Thus, the PKC/NFKBIA/NF-κB-dependent anti-apoptotic signalling deciphered, here, may represent at least one functional pathway crucial in the maintenance of a definite marker-expressing, therapeutically resistant and prognostically relevant stem-like TICs in human prostate cancers. Finally, our screening design to test for candidate small molecule inhibitors that target TICs in a cell type specific manner may represent an interesting approach for other human prostate tumour models and tumours of other organ systems. Institutional protocols All animal experiments and human patient specimen-procurement were performed in accordance with protocols approved by our Institutional Animal Care and Use Committee and Institutional Review Board following National Institutes of Health guidelines for animal welfare and human subject research. Prostate tumours and tumour cell-derived spheres Prostate tumour tissues were minced with Miltex stainless steel disposable safety scalpels in serum-free medium (serum-free insulin rich N 2 medium [55] or human embryonic stem cell (HES) medium [56] ), supplemented with 2% B-27 supplement without vitamin A (Invitrogen), 20 ng ml −1 FGF2 (R&D Systems) and 20 ng ml −1 EGF (R&D Systems). Tissue was digested with 0.5 mg ml −1 collagenase Type 1A (Sigma) and 100 U ml −1 RNase-free DNase (Promega) to reduce cell clumping during tissue dissociation for 90 min at 37 °C with constant agitation. Dissociated tissue was passed through 100 μm cell strainer filter (BD Falcon). The resulting cells were pelleted at 800 g using the Eppendorf centrifuge 5810, and the pellet was treated with 1× conc of BD Pharm Lyse lysing buffer (BD BioSciences) for 1 min to deplete erythrocytes followed by neutralization in phosphate buffered saline. Live cell numbers were determined as a function of trypan blue exclusion. The cells were pelleted as above, washed and plated for sphere-formation with N 2 medium, while similar results were obtained with the human embryonic stem cell medium at a cell density of 40–80×10 6 cells per 15 ml medium (unless stated otherwise) in nonadherent 10-cm dishes (Costar). For determining sphere-forming efficiency, dissociated total tumour cells or the primary sphere-derived cells (following Acutase treatment and trituration) were plated in 6–12 well nonadherent plates at the desired cell densities. The medium was changed daily along with growth factor supplementation, and the spheres were collected at the specified time points following gravity-based sedimentation and/or low-speed centrifugation to remove any remaining single cells. Spheres were then washed once with phosphate buffer saline, followed by gentle resuspension in cell detachment solution (Accutase/Accumax, Innovative Cell Technology; with the aid of a pipette tip) and constant trituration (twice for every 3–5 min) for at least 20 min to obtain single cells. The dissociated single cells of the primary spheres were washed at least three times with the N 2 medium and then plated for sequential sphere-formation for an additional 3–6 days or transplanted immediately into mice at OT or SC sites for tumour-initiation assays. Western blotting Immunoblotting was performed with whole cell lysates as previously described, [57] with the following modifications. The cell lysates (200 μg per well) were separated in 4–12% Bis–Tris NuPAGE gel (Invitrogen) using the i-Blot gel transfer system essentially using the reagents and the materials supplied by the manufacturer (Invitrogen). All the washings were for 15 min with the phosphate buffer saline containing 0.1% Tween-20 (Fisher Scientific); the last wash before chemical detection of the western reaction was without Tween-20. Primary antibody binding was visualized by chemiluminescence derived from the Super Signal West Pico substrate (Pierce) with the HRP-secondary antibody conjugate (Pierce). Chemiluminescence was captured on Kodak Biomax MR Film (Kodak). Prospective purification by FACS Dissociated tumour or sphere cells were sieved through nylon cell strainers (70 μm; BD Falcon) and pelleted in aliquots of >10 6 cells for BSA blocking in FACS buffer, followed by incubation with various conjugated primary antibodies at the manufacturers' suggested and/or pre-optimized concentrations for 90 min at 4 °C in the dark with the same buffer in a final volume of 100–500 μl. The cell samples were then pelleted, the supernatant aspirated and then washed twice with FACS buffer without antibodies, and maintained in the dark on ice until subjected to FACS (for a maximum of 1 h). Flow cytometric data acquisition and sorting were carried out using a stream-in-air FACS Vantage DiVa cell sorter (BD Biosciences) equipped with three lasers (488, 633, 360 nm) and optics for seven-color data acquisition. DiVa software version 4.1.2 was used to acquire and sort cells positive for Alexa 488+, Alexa 647+, APC+, FITC+ and PE+. Instrument performance was verified before acquisition using standard fluorescent microparticles (SPHERO Rainbow Fluorescent Particles, RFP 30-5A, Spherotech). Fluorescent detector voltages were set so that the unstained cells were on scale, and compensation was calculated manually in the DiVa software using single-stained controls. Data analysis was performed using FlowJo software version 8.7.3 (Tree Star). Greater than 30,000 events were collected and gated to include live cells (forward scatter versus side scatter) and exclude doublets (forward scatter area versus forward scatter height). Singlet-gated unstained cells were used to draw gates to identify Alexa 488+, Alexa 647+, APC+, FITC+ and PE+ single-positive ( Supplementary Figs S2 and S3a–c ) or double-positive ( Supplementary Fig. S3d–f ) populations depending on the stain used. Unless stated otherwise, for sorting and analysis of these triple-marker-positive (Alexa 488 conjugated TRA-1-60+/PE conjugated CD151+/Alexa 647 conjugated CD166+) cells, we selected the brightly triple-marker-positive cell populations (high expressors; Compare Supplementary Fig. S4a,b ) and excluded cells with low expression (total expressors; Supplementary Fig. S4a–c ) of the three markers. Strategies to gate for triple-negatives are also depicted ( Supplementary Fig. S4d ). Percent sphere-formation was routinely greater in the high expressors than in the low expressors of these triple-markers. By using alternative fluorochrome(s) conjugated to the same primary antibodies (such as Alexa 647 conjugated anti-TRA-1-60 or anti-CD-151 antibodies and PE conjugated anti-CD166 antibody) the specificity of antigen expression on the tumour cells was verified. Microarray Total RNA was isolated from freshly snap-frozen tumour cells, spheres and the prospectively purified cells using TRIzol and suggested protocol (Invitrogen). All the samples of a given set were processed in parallel for total RNA extraction to avoid batch variations. Total RNA samples were processed by the SKI Genomics Core Facility for mRNA and miRNA analysis using standard protocols. Gene expression analysis was performed using the Illumina Human Ref6V2 bead chip arrays. Analysis of miRNA expression was performed using the Agilent miRNA microarrays (Human_miRNAV1, Agilent). Scanned images were processed with the Illumina bead studio program to define levels of gene expression. These raw data were further processed using the Bioconductor Lumi package to normalize (quantile) and log-transform the data. For miRNA analysis, scanned images were processed with the Agilent feature extraction program, which provided raw signal values for each miRNA (Gene signals). The data were normalized using Variance Stabilization Normalization from the Bioconductor VSN package and log-transformed. Data computation for both mRNA and miRNA are as follows: to compute differentially expressed 'genes,' the Bioconductor LIMMA packages was used for a corrected t -test using an empirical Bayes method to compute variance correction and P values. To adjust for multiple testing, the False Discovery Rate method was used. Fold changes were converted to the signed real space convention; fold changes less than zero are the minus of the reciprocals; that is, −2 is really 1/2. Average signal levels are the averages of the log signal transformed back into real space. Genes were annotated for their associated biological processes and molecular functions by Gene Ontology project ( http://www.geneontology.org/index.shtml ). Comprehensive functional annotation of the gene sets was carried out with the Database for Annotation, Visualization and Integrated Discovery (DAVID) 2008 program ( http://david.abcc.ncifcrf.gov/ ). The miRNA targets and expression were determined using publicly available databases ( http://www.targetscan.org/ and/or http://www.microrna.org/microrna/home.do ). The miRNA function in gene and pathway regulation was obtained using ARGONAUTE 2- database ( http://www.ma.uni-heidelberg.de/apps/zmf/mirwalk/ ). Both the RNA and miRNA expression data sets are deposited in GEO ( http://www.ncbi.nlm.nih.gov/geo/ ) with accession numbers GSE25690 and GSE25691 , respectively. Screening of stem-like TICs with small molecule inhibitors Inhibitors of various signalling pathways, namely, Met receptor kinase (PHA 665752 (PHA), Tocris BioScience), NF-κB signalling (481407 compound (Calbiochem); parthenolide (TocrisBioScience), celastrol (TocrisBioScience), BAY11-7082 (Calbiochem)), PKC signalling (Staurosporine (Calbiochem)), proteasomes (MG132 (Calbiochem)), MAP kinase (U0126 (Promega)), PI3 Kinase (LY 294002 (Calbiochem)), mTOR (Rapamycin (Sigma)), Hedgehog signalling (Cyclopamine (Sigma)) or Notch signalling (DAPT: N -[ N -(3,5-difluorophenacetyl- L -alanyl)]-S-phenylglycine t-butyl ester (Sigma)), were administered for 16 h to total tumour cells about 60 h post-initiation of primary spheres. The primary spheres were collected, washed twice with the same growth medium depleted of the inhibitors and finally once with phosphate-buffered saline. The spheres were then dissociated into single cells as described above. Dimethylsulphoxide-treated sample served as control for the inhibitor-treated ones. For testing the effect of various small molecule inhibitors on primary sphere-formation, we used at least 100,000 total tumour cells isolated from different human prostate tumour xenografts as described. To follow the subsequent effects of the same inhibitors on secondary sphere-formation, we used at least 5,000, 25,000 and 10,000 primary sphere cells derived from human prostate CWR22 OT-tumours, parent DU-145 SC-/PC-82 OT-tumours and the prospectively purified TRA-1-60-positive cell-derived DU-145 SC- /PC-82 OT-tumours, respectively. To investigate the tumour-initiation ability following the above inhibitor treatments, 2500–5000 primary sphere cells were transplanted as indicated. Additional experimental details are described in the Supplementary Information . Accession codes. Expression data sets were deposited in GEO under accession numbers GSE25690 and GSE25691 . How to cite this article: Rajasekhar, V. K. et al . Tumour-initiating stem-like cells in human prostate cancer exhibit increased NF-κB signalling. Nat. Commun. 2:162 doi: 10.1038/ncomms1159 (2011).